Double thermoelectric power factor of a 2D electron system 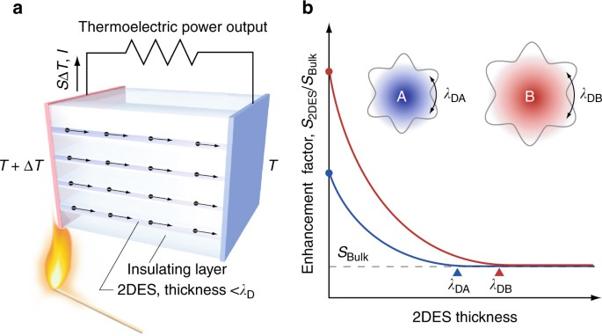Fig. 1 Thermoelectric effect of a 2D electron system.aSchematic illustration of thermoelectric Seebeck effect in a 2DES. A thermoelectric power output (S·ΔT·I) can be obtained when ΔTis introduced.bThe hypothesis that a 2DES with longer de Broglie wavelength (λD) shows a larger enhanced factor of thermopower Two-dimensional electron systems have attracted attention as thermoelectric materials, which can directly convert waste heat into electricity. It has been theoretically predicted that thermoelectric power factor can be largely enhanced when the two-dimensional electron layer is far narrower than the de Broglie wavelength. Although many studies have been made, the effectiveness has not been experimentally clarified thus far. Here we experimentally clarify that an enhanced two-dimensionality is efficient to enhance thermoelectric power factor. We fabricated superlattices of [ N unit cell SrTi 1− x Nb x O 3 |11 unit cell SrTiO 3 ] 10 —there are two different de Broglie wavelength in the SrTi 1− x Nb x O 3 system. The maximum power factor of the superlattice composed of the longer de Broglie wavelength SrTi 1− x Nb x O 3 exceeded ∼ 5 mW m −1 K −2 , which doubles the value of optimized bulk SrTi 1− x Nb x O 3 . The present approach—use of longer de Broglie wavelength—is epoch-making and is fruitful to design good thermoelectric materials showing high power factor. Currently, more than 60% of the energy produced from fossil fuels is lost as waste heat. Thermoelectric energy conversion, which is the process where waste heat is transformed into electricity by the Seebeck effect, is attracting attention as a potential energy harvesting technology [1] , [2] , [3] , [4] . The performance of thermoelectric materials is generally evaluated in terms of a dimensionless figure of merit, 
    ZT = S^2 ·σ· T ·κ ^ - 1,
 (1) where Z is the figure of merit, T is the absolute temperature, S is the thermopower (Seebeck coefficient), σ is the electrical conductivity, and κ is the sum of the electronic ( κ ele ) and lattice thermal conductivities ( κ lat ) of a thermoelectric material. There are two strategies to improve ZT of a thermoelectric material. One is to reduce κ lat . Recently, state-of-the-art nanostructuring techniques have reduced κ lat significantly through phonon scattering by nanosized structural defects [5] , [6] , [7] , [8] . Such techniques have realized high-performance thermoelectric materials with a large ZT of 1.5−2. The other strategy is an enhancement of the product S 2 ∙ σ , which is called power factor (PF). However, it is extremely difficult to enhance PF due to the trade-off relationship between S and the carrier concentration ( n ). Therefore, PF has a local maximum value in three-dimensional (3D) bulk systems. In a two-dimensional electron system (2DES) such as metal/insulator superlattices, electron carriers are confined within a thin layer (thickness thinner than the de Broglie wavelength, λ D ). 2DES is an efficient strategy to achieve an enhanced PF. The effectiveness of 2DES was theoretically predicted by Hicks and Dresselhaus [9] ; 2DES in extremely narrow layers exhibits an enhanced S without reducing σ because the density of states (DOS) near the bottom of the conduction band increases as the 2DES layer thickness decreases. These layers are narrower than the λ D , 
    λ _D = h/√(3 · m^∗· k_B· T),
 (2) where h , m *, and k B are Planck’s constant, effective mass of conductive electron or hole, and Boltzmann constant, respectively [9] , [10] , [11] , [12] , [13] . Many experimental studies have been made to clarify the effectiveness of 2DES to enhance PF using PbTe/Pb 1− x Eu x Te multiple-quantum-well [10] , electron-doped SrTiO 3 -based superlattices [14] , [15] , SiGe-based superlattices [16] , [17] , and Bi 2 Te 3 -based superlattices [18] . These 2DES layers showed enhanced S . However, total enhancement of PF was very small because of the insulator layer thickness. Thus, the effectiveness of 2DES has not been experimentally clarified thus far. Here we experimentally clarify that an enhanced two-dimensionality is efficient to improve thermoelectric PF. 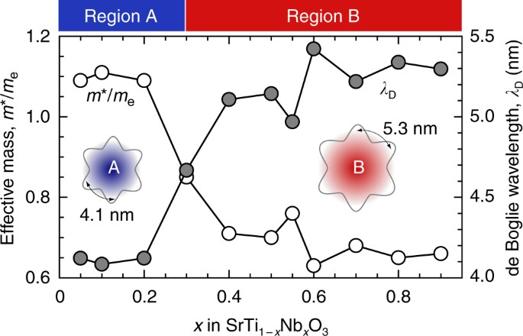Fig. 2 SrTiO3–SrNbO3solid solution: a model system having two differentλD.x-dependent effective mass (m*/me, white symbols) andλD(gray symbols) for SrTi1 −xNbxO3solid solutions.m*/meexerts a decreasing tendency withx, resulting in an increasedλD. Sharp changes in bothm*/meandλDare detected aroundx= 0.3 due to the conduction band transition from Ti 3dto Nb 4d. The properties of SrTi1 −xNbxO3solid solutions can be divided into two regions based on the conduction bands (Ti 3d→ region A and Nb 4d→ region B). Inset: schematic illustrations of conduction electrons at regions A and B. At region B,λDis∼5.3 nm, while it is∼4.1 nm at region A We fabricated superlattices of [ N unit cell SrTi 1− x Nb x O 3 |11 unit cell SrTiO 3 ] 10 —there are two different de Broglie wavelength in the SrTi 1− x Nb x O 3 system. The maximum PF of the superlattice composed of the longer de Broglie wavelength SrTi 1− x Nb x O 3 exceeded ~5 mW m −1 K −2 , which doubles the value of optimized bulk SrTi 1− x Nb x O 3 . The present approach—use of longer de Broglie wavelength—is epoch-making and is fruitful to design good thermoelectric materials showing high PF. Hypothesis In order to enhance total PF of 2DES, two-dimensionality should be enhanced. Use of longer λ D should be effective if the electron carriers are confined within a defined thickness layer (Fig. 1 ). Very recently, we observed a steep decrease in m */ m e at x ~ 0.3 in SrTiO 3 –SrNbO 3 solid solution system, SrTi 1− x Nb x O 3 ( x is ranging from 0.05 to 0.9; Fig. 2 ) [19] . The ratio x of SrTi 1− x Nb x O 3 can be divided into two regions, region A ( x is <0.3) and region B ( x is >0.3). The origin of the two regions is most likely due to the difference in the overlap population between the Ti 3 d and Nb 4 d orbitals ( r Ti3 d is 48.9 pm and r Nb4 d is 74.7 pm) [20] . We calculated λ D values of SrTi 1− x Nb x O 3 using the Eq. (2). The λ D value in region B is ~5.3 nm, which is 27% longer than that in region A (~4.1 nm). One can expect that S -enhancement factor in region B is much higher than that in region A because of higher two-dimensionality. Therefore, we hypothesized that SrTi 1− x Nb x O 3 -based 2DES can be used to clarify the effectiveness of 2DES to enhance PF experimentally. Fig. 1 Thermoelectric effect of a 2D electron system. a Schematic illustration of thermoelectric Seebeck effect in a 2DES. A thermoelectric power output ( S ·Δ T · I ) can be obtained when Δ T is introduced. b The hypothesis that a 2DES with longer de Broglie wavelength ( λ D ) shows a larger enhanced factor of thermopower Full size image Fig. 2 SrTiO 3 –SrNbO 3 solid solution: a model system having two different λ D . x -dependent effective mass ( m */ m e , white symbols) and λ D (gray symbols) for SrTi 1 − x Nb x O 3 solid solutions. m */ m e exerts a decreasing tendency with x , resulting in an increased λ D . Sharp changes in both m */ m e and λ D are detected around x = 0.3 due to the conduction band transition from Ti 3 d to Nb 4 d . The properties of SrTi 1 − x Nb x O 3 solid solutions can be divided into two regions based on the conduction bands (Ti 3 d → region A and Nb 4 d → region B). Inset: schematic illustrations of conduction electrons at regions A and B. At region B, λ D is ∼ 5.3 nm, while it is ∼ 4.1 nm at region A Full size image We fabricated [ N uc SrTi 1− x Nb x O 3 |11 uc SrTiO 3 ] 10 superlattices ( N is ranging from 1 to 12, x is ranging from 0.2 to 0.9) by a pulsed laser deposition (PLD) technique on insulating (001) LaAlO 3 (pseudo-cubic perovskite, the lattice parameter, a is 3.79 Å) single-crystal substrates using dense ceramic disks of a SrTiO 3 –SrNbO 3 mixture and SrTiO 3 single crystal as the targets. The thicknesses of different layers were monitored in situ using the intensity oscillation of the reflection high-energy electron diffraction (RHEED) spots. (See Experimental Section.) High-resolution X-ray diffraction (XRD) measurements revealed that the resultant superlattices were heteroepitaxially grown on (001) LaAlO 3 with cube-on-cube epitaxial relationship with superlattice structure. Atomically smooth surfaces with stepped and terraced structure were observed by an atomic force microscopy (AFM). 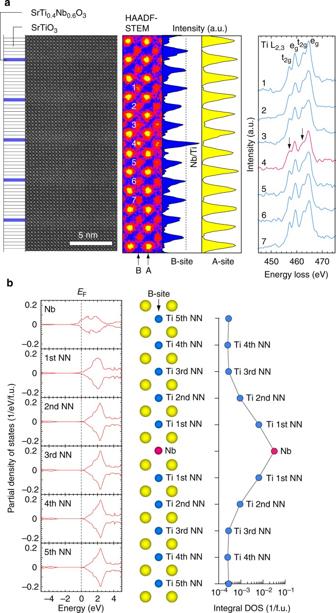Fig. 3 Experimental and theoretical analyses of the 2DES.aCross-sectional HAADF-STEM image of the [1 uc SrTi0.4Nb0.6O3|11 uc SrTiO3]10superlattice. Layer stacking sequence is also shown. Rather bright bands are seen near each SrTi0.4Nb0.6O3layer. In the magnified image, the #4 atom in the B-site column is brighter than the nearby atoms, whereas no obvious difference is observed in the A-site column. EELS spectrum of #4 is broader than that of nearby atoms, indicating the coexistence of Ti4+/Ti3+in the SrTi0.4Nb0.6O3layers.bThe calculated partial DOS of Nb 4dor Ti 3din the [1 uc SrNbO3|10 uc SrTiO3] superlattice. The Fermi energy (EF) is located on the higher-energy side of the conduction band minimum for the first and second nearest neighbor (Ti first NN and Ti second NN). SrTiO3layers together with 1 uc SrNbO3layer (Nb) suggest that the electron carriers can seep from the SrTi1 −xNbxO3layers into the SrTiO3layers Microstructure and electronic structure Figure 3a summarizes the atomic arrangements of the [1 uc SrTi 0.4 Nb 0.6 O 3 |11 uc SrTiO 3 ] 10 superlattice. Rather bright bands are observed near each SrTi 0.4 Nb 0.6 O 3 layer in the Cs-corrected high-angle annular dark-field scanning transmission electron microscopy (HAADF-STEM) image. In the magnified image, the #4 atom in the B-site column is brighter than the nearby atoms. However, there is no obvious difference in the A-site column, indicating Nb substitution occurs for the #4 atom in the B-site column. The electron energy loss spectroscopy signal of #4 is broader than that of the nearby atoms, implying the coexistence of Ti 4+ /Ti 3+ in the SrTi 0.4 Nb 0.6 O 3 layers [21] . Therefore, in our superlattice fabrication, Nb ions are successfully confined into 1 uc of SrTi 0.4 Nb 0.6 O 3 layers [22] . Fig. 3 Experimental and theoretical analyses of the 2DES. a Cross-sectional HAADF-STEM image of the [1 uc SrTi 0.4 Nb 0.6 O 3 |11 uc SrTiO 3 ] 10 superlattice. Layer stacking sequence is also shown. Rather bright bands are seen near each SrTi 0.4 Nb 0.6 O 3 layer. In the magnified image, the #4 atom in the B-site column is brighter than the nearby atoms, whereas no obvious difference is observed in the A-site column. EELS spectrum of #4 is broader than that of nearby atoms, indicating the coexistence of Ti 4+ /Ti 3+ in the SrTi 0.4 Nb 0.6 O 3 layers. b The calculated partial DOS of Nb 4 d or Ti 3 d in the [1 uc SrNbO 3 |10 uc SrTiO 3 ] superlattice. The Fermi energy ( E F ) is located on the higher-energy side of the conduction band minimum for the first and second nearest neighbor (Ti first NN and Ti second NN). SrTiO 3 layers together with 1 uc SrNbO 3 layer (Nb) suggest that the electron carriers can seep from the SrTi 1 − x Nb x O 3 layers into the SrTiO 3 layers Full size image In order to clarify the 2DES formation, the electronic band structures of the [1 uc SrNbO 3 |10 uc SrTiO 3 ] superlattices were calculated based on the projector-augmented wave (PAW) method (Fig. 3b ). The E F is located on the higher-energy side of the conduction band minimum for the first and second nearest-neighbor SrTiO 3 layers (Ti first NN and Ti second NN) together with the 1 uc SrNbO 3 layer (Nb). The electron carriers can seep from the SrNbO 3 layers into the SrTiO 3 layer. Delugas et al. [23] have also predicted theoretically that for lower Nb substituted samples, it is much easier for the electrons, especially in the d xz and d yz bands, to spread out to the neighboring SrTiO 3 layers, reducing the two-dimensionality. However, as the Nb content increases, the minimum thickness of the barrier layer may be reduced to 5 uc in the SrNbO 3 case. There is no doubt that the electron diffusion cannot be removed thoroughly in superlattice structure, but diffusion effects can be effectively suppressed by the high Nb substitution. From the band calculation, 2DES in our work is mainly confined to the 1 uc SrTi 1− x Nb x O 3 layers and should contribute to the S enhancement. In order to further confirm the superlattice structure, we measured the κ of the [1 uc SrTi 0.4 Nb 0.6 O 3 |11 uc SrTiO 3 ] 10 superlattice along the cross-plane direction by time-domain thermal reflectance (TDTR) method. The total κ could be suppressed to ~3.3 W m −1 K −1 , similar to the minimum value of CaTiO 3 /SrTiO 3 -based superlattices ( κ ~ 3.2 W m −1 K −1 ) reported by Ravichandran et al. [24] . From these results, we judged that our [ N uc SrTi 1− x Nb x O 3 |11 uc SrTiO 3 ] 10 superlattices ( N is ranging from 1 to 12, x is ranging from 0.2 to 0.9) are appropriate for us to clarify the effectiveness of 2DES to enhance PF. Thermoelectric properties The electrical conductivity ( σ ), carrier concentration ( n ), and Hall mobility ( μ Hall ) of the superlattices were measured at room temperature by a conventional d.c. four-probe method with a van der Pauw geometry. S was measured at room temperature by creating a temperature difference (Δ T ) of ~4 K across the film using two Peltier devices. 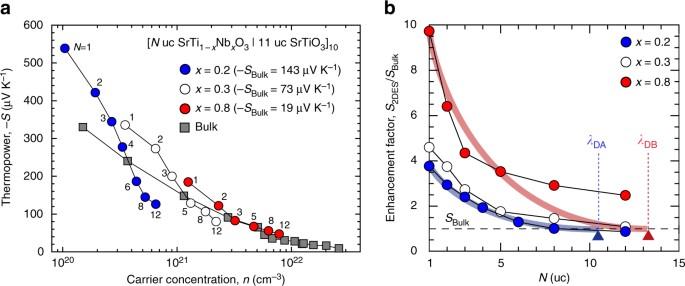Fig. 4 Two-dimensionality of 2DES: a key to enhance thermopower.aPlots of thermopower of the 2DESs, [Nuc SrTi1 −xNbxO3|11 uc SrTiO3]10superlattices (x= 0.2, 0.3, and 0.8), versus the carrier concentration (n). Compared to bulk values (gray squares), all the 2DESs show an enhanced −SasNis reduced under 3 uc.bEnhancement factors in –S(S2DES/SBulk) for three sets of 2DESs. Forx= 0.2 and 0.3 2DESs, the highestS2DES/SBulkvalues are obtained atN= 1, which are 4 and 5, respectively, while that ofx= 0.8 can reach 10 Figure 4a summarizes the n -dependent S of [ N uc SrTi 1− x Nb x O 3 |11 uc SrTiO 3 ] 10 superlattices ( N is ranging from 1 to 12, x = 0.2, 0.3, and 0.8) along with bulk (~100-nm-thick SrTi 1− x Nb x O 3 films, x = 0.2, 0.3, and 0.8, respectively) values for comparison. The bulk S for x = 0.2 was −143 μV K −1 , x = 0.3 was −73 μV K −1 , and x = 0.8 was −19 μV K −1 . The n value was measured based on the total thickness of the 2DES, which includes the insulating SrTiO 3 layers. All the 2DES samples show enhanced thermopower (− S ) with a reduced N . Compared to the bulk samples at a similar n , a much higher − S is observed in superlattices as N is reduced below 3 uc. Fig. 4 Two-dimensionality of 2DES: a key to enhance thermopower. a Plots of thermopower of the 2DESs, [ N uc SrTi 1 − x Nb x O 3 |11 uc SrTiO 3 ] 10 superlattices ( x = 0.2, 0.3, and 0.8), versus the carrier concentration ( n ). Compared to bulk values (gray squares), all the 2DESs show an enhanced − S as N is reduced under 3 uc. b Enhancement factors in – S ( S 2DES / S Bulk ) for three sets of 2DESs. For x = 0.2 and 0.3 2DESs, the highest S 2DES / S Bulk values are obtained at N = 1, which are 4 and 5, respectively, while that of x = 0.8 can reach 10 Full size image To confirm the increasing two-dimensionality with x , the S -enhancement factors ( S 2DES / S Bulk ) were plotted versus the N values (Fig. 4b ). For 2DES with x = 0.2 and 0.3, the highest S 2DES / S Bulk values are around 4 and 5, respectively, whereas that for the x = 0.8 counterpart is ~10. As hypothesized, the enhanced S 2DES / S Bulk should stem from the increasing λ D with x . In our experiment, S 2DES / S Bulk for the x = 0.2 and 0.3 2DESs are saturated around 11 uc, which is consistent with λ D in region A (~4.2 nm indicated by dashed line λ DA ). As λ D increases in region B, the saturation position for the x = 0.8 2DES has a thickness larger than the λ D (~5.2 nm indicated by dashed line λ DB ). As a result, a significantly enhanced two-dimensionality is achieved in the x > 0.3 region B, which fits well with our hypothesis and suggests that region B has the potential to further enhance the thermoelectric PF. Based on the conclusions above, we have enhanced the thermoelectric PF in [1 uc SrTi 1− x Nb x O 3 |11 uc SrTiO 3 ] 10 superlattices by adjusting x between 0.2 and 0.9. 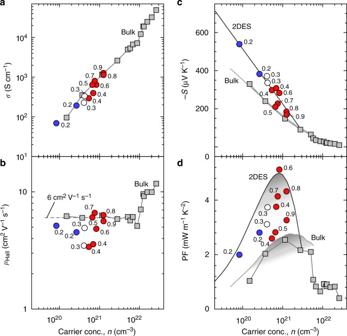Fig. 5 Double enhancement of the thermoelectric power factor in a 2DES. Carrier concentration dependences ofaelectrical conductivity (σ),bHall mobility (μHall),cthermopower (−S), anddpower factor [PF (S2·σ)] of [1 uc SrTi1 −xNbxO3| 11 uc SrTiO3]102DESs (xis ranging from 0.2 to 0.9) at room temperature. Similar to the trends in the bulk values,σincreases almost linearly withn.μHallfor lowerxsamples (x≤ 0.5) fluctuates around 3–5 cm2V−1s−1, while that for higherxones (x≥ 0.6) is ~6 cm2V−1s−1. Slope of –Sversus lognfor bulk SrTi1 −xNbxO3is –198 μV K−1, which is∼1.5 times lower than –300 μV K−1for the 2DESs. Double enhancement of PF is seen inx= 0.6 (5.1 mW m−1K−2atn∼8 × 1020cm−3). Since the PF values are scattered due to the rather large distribution ofμHall(3–6 cm2V−1s−1), we calculated PFs using the relationship betweenSandn(c) at constantμHall(6 cm2V−1s−1). The optimized PF of the 2DES should be ~5 mW m−1K−2atn∼8 × 1020cm−3, which doubles that of bulk SrTi1 −xNbxO3(PF∼2.5 mW m−1K−2atn∼2 × 1021cm−3) Figure 5 summarizes the n dependences of the thermoelectric properties of [1 uc SrTi 1− x Nb x O 3 |11 uc SrTiO 3 ] 10 superlattices at room temperature along with the reported bulk values for comparison [19] . Following the bulk values, σ increases almost linearly with n (Fig. 5a ), indicating that n dominates σ . In the SrTi 1− x Nb x O 3 system, carriers are mostly due to Nb substitution. The high n also induces a highly Nb substituted region with a superiority in σ . However, σ for the superlattices remains lower than the bulk value due to the coexistence of 11 uc SrTiO 3 insulating layers. Fig. 5 Double enhancement of the thermoelectric power factor in a 2DES. Carrier concentration dependences of a electrical conductivity ( σ ), b Hall mobility ( μ Hall ), c thermopower (− S ), and d power factor [PF ( S 2 · σ )] of [1 uc SrTi 1 − x Nb x O 3 | 11 uc SrTiO 3 ] 10 2DESs ( x is ranging from 0.2 to 0.9) at room temperature. Similar to the trends in the bulk values, σ increases almost linearly with n . μ Hall for lower x samples ( x ≤ 0.5) fluctuates around 3–5 cm 2 V −1 s −1 , while that for higher x ones ( x ≥ 0.6) is ~6 cm 2 V −1 s −1 . Slope of – S versus log n for bulk SrTi 1 − x Nb x O 3 is –198 μV K −1 , which is ∼ 1.5 times lower than –300 μV K −1 for the 2DESs. Double enhancement of PF is seen in x = 0.6 (5.1 mW m −1 K −2 at n ∼ 8 × 10 20 cm −3 ). Since the PF values are scattered due to the rather large distribution of μ Hall (3–6 cm 2 V −1 s −1 ), we calculated PFs using the relationship between S and n (c) at constant μ Hall (6 cm 2 V −1 s −1 ). The optimized PF of the 2DES should be ~5 mW m −1 K −2 at n ∼ 8 × 10 20 cm −3 , which doubles that of bulk SrTi 1 − x Nb x O 3 (PF ∼ 2.5 mW m −1 K −2 at n ∼ 2 × 10 21 cm −3 ) Full size image μ Hall for lower x of 2DESs ( x ≤ 0.5) fluctuates around 3–5 cm 2 V −1 s −1 , while for higher x 2DESs ( x ≥ 0.6) values are ~6 cm 2 V −1 s −1 (Fig. 5b ). Usually, μ Hall is controlled by the conduction band of materials along with the effects of crystal defects such as impurities and grain boundaries. In the bulk samples, μ Hall sharply increases due to the transition of the conduction band from Ti 3 d to Nb 4 d as x increases into the highly Nb substituted region [19] . This pattern is also observed in the superlattice counterparts. A higher μ Hall (≥6 cm 2 V −1 s −1 ) is observed in samples with x ≥ 0.6 than that for x ≤ 0.5 (3–5 cm 2 V −1 s −1 ). Compared to the bulk samples, all the superlattices exert a much lower μ Hall , which may result from an insufficient crystal quality or electron diffusion into the pure SrTiO 3 barrier layers. Regardless, a conduction band transition from Ti 3 d to Nb 4 d is recognized in our superlattice systems. Due to the high overlapping population of the Nb 4 d orbital, a superior electron transport property is realized in higher x of 2DES. Figure 5c plots the S values for all the superlattices versus n along with the reported bulk values [19] . The solid line depicts the overall tendency. In the diagram, the superlattices have a significantly enhanced – S compared to bulk samples at similar n values. As indicated by the solid lines, the experimental points for 2DES and bulk show different slopes of –300 and –200 μV K −1 per decade, respectively. The relationship between – S and n eff can be expressed by Eq. (3) 
    - S = - k_B/e·ln 10· A·( log n + B),
 (3) where k B is the Boltzmann constant and e is an electron charge. A and B are the parameters that depend on the type of materials and their electronic band structures. Bulk shows a 3D electronic band structure with a parabolic shaped DOS near E F , where the A value = 1 and the slope reflects a constant value of − k B / e ·ln10 (−198 μV K −1 ). On the other hand, the slope of the 2DESs may reach −300 μV K −1 per decade, indicating that the A value = 1.5. Therefore, the 2DESs work well to enhance the S even for the whole superlattice, including SrTiO 3 insulating layers. Finally, we calculated PF of the [1 uc SrTi 1− x Nb x O 3 |11 uc SrTiO 3 ] 10 superlattices ( x is ranging from 0.2 to 0.9) using the observed S and σ values (Fig. 5d ). PF is doubly enhanced for x = 0.6 (5.1 mW m −1 K −2 at n ~ 8 × 10 20 cm −3 ). Since the PF values are scattered due to the rather large distribution of μ Hall (3–6 cm 2 V −1 s −1 ), we calculated PFs using the relationship between S and n (c) at constant μ Hall (6 cm 2 V −1 s −1 ). The optimized PF of the 2DES should be ~5 mW m −1 K −2 at n ~ 8 × 10 20 cm −3 , which doubles that of bulk SrTi 1− x Nb x O 3 (PF ~ 2.5 mW m −1 K −2 at n ~ 2 × 10 21 cm −3 ). The present 2DES, [1 uc SrTi 1− x Nb x O 3 |11 uc SrTiO 3 ] 10 superlattices ( x is ranging from 0.2 to 0.9), has several merits to enhance PF as compared with other 2DESs such as PbTe/Pb 1− x Eu x Te multiple-quantum-well [10] , SiGe-based superlattices [16] , [17] , and Bi 2 Te 3 -based superlattices [18] , which are already commercialized thermoelectric materials. This is because SrTi 1− x Nb x O 3 can be deposited with 1 uc layer accuracy by PLD. Therefore, we can easily reduce the 2DEG thickness to ~0.4 nm (1 uc layer). Further, there are two different λ D in SrTi 1− x Nb x O 3 ; ~4.1 nm in the low conducting region and ~5.3 nm in the high conducting region. For enhancing PF, both S and σ play important roles. The present research implies that high conducting region is effective to enhance the thermoelectric PF in the 2DES. Herein highly Nb substitution are revealed to have the coexistence of both a high electron transport (high n and μ Hall ) and a high two-dimensionality (large λ D ). In summary, we have experimentally clarified that an enhanced two-dimensionality of 2DES is efficient to improve thermoelectric PF. We measured the thermoelectric properties of 2DESs [ N uc SrTi 1− x Nb x O 3 |11 uc SrTiO 3 ] 10 superlattices ( N is ranging from 1 to 12, x is ranging from 0.2 to 0.9) because there are two different λ D in this 2DES ( x > 0.3: λ D ~5.3 nm; x < 0.3: λ D ~4.1 nm). The S -enhancement factor S 2DES / S Bulk of the 2DES ( N = 1) for x > 0.3 were ~10, whereas those for x < 0.3 were 4–5. Maximum PF of the 2DES ( N = 1, x = 0.6) exceeded ~5 mW m −1 K −2 , which doubles the value of optimized bulk SrTi 1− x Nb x O 3 (PF ~ 2.5 mW m −1 K −2 ). The present 2DES approach—use of longer λ D —is epoch-making and is fruitful to design good thermoelectric materials showing high PF. Fabrication and analyses of the 2DESs A series of superlattices with the chemical formula of [ N uc SrTi 1− x Nb x O 3 | 11 uc SrTiO 3 ] 10 ( N is ranging from 1 to 12, x is ranging from 0.2 to 0.9) were fabricated by a PLD technique using dense ceramic disks of a SrTiO 3 –SrNbO 3 mixture and a SrTiO 3 single crystal as the targets. The substrate was insulating (001) LaAlO 3 (pseudo-cubic perovskite, lattice parameter, a is 3.79 Å, the surface area: 1 cm × 1 cm). The growth conditions were precisely controlled; the substrate temperature was 900 °C, the oxygen pressure was ~10 −4 Pa, and the laser fluence was ~1.2 J cm −2 per pulse. The thicknesses of different layers were monitored in situ using the intensity oscillation of the RHEED spots. Details of our PLD growth process of the superlattices are reported elsewhere [14] , [25] . Crystallographic analyses of the resultant superlattices were performed by XRD (Cu Kα 1 , ATX-G, Rigaku Co.), AFM (Nanocute, Hitachi Hi-Tech), and STEM (200 keV, JEM-ARM 200CF, JEOL Co. Ltd). TEM samples were fabricated using a cryo ion slicer (IB-09060CIS, JEOL Co. Ltd). HAADF images were taken with the detection angle of 68–280 mrad. Electron energy loss spectra were acquired in STEM mode with the energy resolution of 0.8 eV. Measurements of the thermoelectric properties of the 2DESs Electrical conductivity ( σ ), carrier concentration ( n ), and Hall mobility ( μ Hall ) were measured at room temperature by a conventional d.c. four-probe method with a van der Pauw geometry. S was measured at room temperature by creating a temperature difference (Δ T ) of ~4 K across the film using two Peltier devices. (Two small thermocouples were used to monitor the actual temperatures of each end of a superlattice.) The thermo-electromotive force (Δ V ) and Δ T were measured simultaneously, and the S values were obtained from the slope of the Δ V –Δ T plots (the correlation coefficient: >0.9999). Cross-plane thermal conductivity ( κ ) was measured by TDTR (Picotherm Co.) method. Mode-locked fiber pulse lasers with 1550 and 775 nm wavelengths were used for heating and measuring, respectively. Both lasers are with the repetition frequency of 20 MHz and pulse duration of 0.4 ps. Before measurement, Mo film with a thickness of 100 nm was first deposited on the surface of the sample as the transducer. During measurement, time-dependent transient thermoreflectance phase signal of Mo transducer was measured, from which κ was further simulated. Time-domain thermoreflectance was measured based on amplified laser systems (5 kHz and ~200 fs centered at 1030 nm). Degenerate pump and probe photons were separated by the cross polarization, and a polarizing filter was employed before the lock-in detection. A mechanical delay stage was used for time scan up to 1.5 ns. Pump to probe intensity ratio was >15, and the size ratio was around 6. Energy band calculation of the 2DES Band structure for the [1 uc SrNbO 3 |10 uc SrTiO 3 ] superlattice was calculated based on the PAW method [26] , as implemented in the VASP code [27] , [28] . We adopted the Heyd–Scuseria–Ernzerhof hybrid functionals [29] , [30] , [31] and a plane-wave cutoff energy of 550 eV. 6 × 6 × 6 and 6 × 6 × 2 k -point meshes were employed in the total-energy evaluations and geometry optimization for the perovskite unit cells of SrTiO 3 and the superlattice cell, respectively. The in-plane lattice constant of the superlattice cell was fixed at the optimized value of SrTiO 3 while the out-of-plane lattice constant and the atomic coordinates were fully relaxed. Data availability The data that support the findings of this study are available from the corresponding authors upon reasonable request.